Tuneable enhancement of the salt and thermal stability of polymeric micelles by cyclized amphiphiles Cyclic molecules provide better stability for their aggregates. Typically in nature, the unique cyclic cell membrane lipids allow thermophilic archaea to inhabit extreme conditions. By mimicking the biological design, the robustness of self-assembled synthetic nanostructures is expected to be improved. Here we report topology effects by cyclized polymeric amphiphiles against their linear counterparts, demonstrating a drastic enhancement in the thermal, as well as salt stability of self-assembled micelles. Furthermore, through coassembly of the linear and cyclic amphiphiles, the stability was successfully tuned for a wide range of temperatures and salt concentrations. The enhanced thermal/salt stability was exploited in a halogen exchange reaction to stimulate the catalytic activity. The mechanism for the enhancement was also investigated. These topology effects by the cyclic amphiphiles offer unprecedented opportunities in polymer materials design unattainable by traditional means. The cyclic form of polymers is often exploited in nature, typically by DNAs [1] , polypeptides [2] , and polysaccharides [3] . Significant functionalities arise from the unique shape [4] , [5] , [6] , [7] , namely topology effects [8] , [9] , especially in relation to their stability. We designed cyclic amphiphilic block copolymers ( Fig. 1 ) (refs 10 , 11 ) that were inspired by the annular structure of the cell membrane lipids of thermophilic archaea, which are monocellular organisms that inhabit high-temperature environments [12] , [13] . The self-assembled micelle formed therefrom exhibited a cloud point ( T c ) more than 40 °C higher than that of the relevant micelle from the linear counterpart ( Fig. 1 ) (ref. 14 ). On the basis of previous reports that the lower critical solution temperature of poly( N -isopropylacrylamide) in a molecularly dispersed state increases modestly by 5 °C upon cyclization [15] , [16] , [17] , we reasoned that the topology effect was amplified by self-assembly to significantly improve the properties of the polymeric materials, which was unattainable through conventional methods. 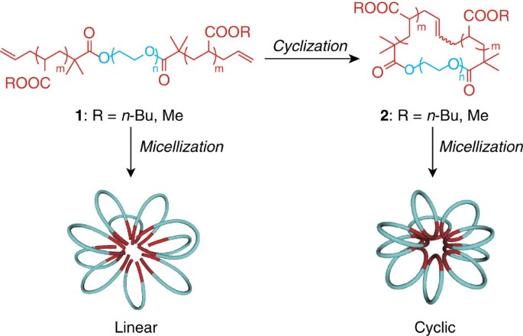Figure 1: Chemical structures of amphiphilic bock copolymers and schematic representation for the formation of micelles. Linear PBA-b-PEO-b-PBA (1a) and PMA-b-PEO-b-PMA (1b,1cand1d) were converted to cyclic PBA-b-PEO (2a) and PMA-b-PEO (2b,2cand2d), respectively. Flower-like micelles were self-assembled from the respective amphiphilic block copolymers. Figure 1: Chemical structures of amphiphilic bock copolymers and schematic representation for the formation of micelles. Linear PBA- b -PEO- b -PBA ( 1a ) and PMA- b -PEO- b -PMA ( 1b , 1c and 1d ) were converted to cyclic PBA- b -PEO ( 2a ) and PMA- b -PEO ( 2b , 2c and 2d ), respectively. Flower-like micelles were self-assembled from the respective amphiphilic block copolymers. Full size image This amplification via self-assembly of a cyclic amphiphile [18] was expected to be expandable to salt stability, which has been hinted by archaea that reside in hypersaline environments [19] . Amphiphiles that form a salt-resistant micelle are applicable not only in detergents used in hard water but also in food and pharmacological processing operations that involve buffer conditions [20] , [21] . The addition of salt has been widely applied to adjust the stability of micelles (for example, from poly(ethylene oxide) (PEO)–poly(propylene oxide) block copolymers, such as Pluronic) [21] , [22] , [23] , [24] . In general, an increase in the salt concentration destabilizes a micelle and lowers the T c . The Hofmeister series empirically shows the effect of the type of anion on the T c (the order of the strength of salting-out: SO 4 2− >Cl − >Br − >NO 3 − >I − >SCN − ). However, the influence of cations is less significant [25] . The aggregation number ( N agg ) of a polymeric amphiphile is also affected [21] , and the influences of salt concentration and temperature on a micellar structure were studied by small-angle neutron scattering [22] . Moreover, a micelle from the Pluronic F-series showed a modest increase in the salting-out concentration ( C s ) by 25–33% when the molecular weight was reduced to approximately one-third [23] . Thus, the improvement in the salt resistance of a micelle by a simple shape transformation of the polymeric surfactant would provide an attractive alternative method with broad applications and avoid extensive chemical modification processes. Herein, we demonstrate the dually tuneable salt and thermal stability of micelles that result from remarkable topology effects of cyclic amphiphiles. The influences of the chemical structures and segment composition on the topology effects were investigated by evaluating the critical micelle concentration (CMC), hydrodynamic diameter ( D h ), D h distribution by the s.d. ( σ ), N agg , second virial coefficient ( A 2 ), T c and C s of the self-assembled micelles. Poly( n -butyl acrylate) (PBA) or poly(methyl acrylate) (PMA) were used for the hydrophobic segments. Because of the smaller size of the monomeric repeating unit in PMA compared with that in PBA, PMA segments longer than their PBA counterparts in the block copolymers were required to form comparable micelles. This approach allowed us to examine the topology effects as a function of the compositional variation of the PMA and PEO segments within an appropriate molecular weight range for the formation of a micelle. The micelles formed from both cyclic PBA- b -PEO and PMA- b -PEO exhibited higher thermal/salt stability under the given experimental conditions. The use of a series of coassemblies of the linear and cyclic amphiphilic block copolymers allowed the micelles’ stability to be tuned over a wide range of salt concentrations and temperatures, which was demonstrated through the experiments on the PBA–PEO block copolymers with the addition of NaCl and MgSO 4 . For practical purposes, such as biological applications, where heating is often inappropriate, the addition of a salt provides an alternative method for controlling the response properties of a micelle. For example, in a drug delivery system, the behaviour of a micellar carrier is programmed for use in a buffer or under physiological conditions, as well as to accommodate drugs that contain organic salt ingredients [24] . Furthermore, the micelle from one of the cyclic copolymers was applied as a catalyst with superior salt and thermal stability for a halogen exchange reaction (Finkelstein reaction) in an aqueous medium and resulted in a significantly enhanced rate. As reactions in water have attracted strong interest for the potential applications in green chemistry [26] , [27] , the present topology-based methodology may serve as a novel approach for the development of innovative materials. Synthesis of block copolymers and formation of micelles Linear PBA- b -PEO- b -PBA and corresponding cyclic PBA- b -PEO were synthesized and characterized according to previously reported protocols [10] . Analogously, linear PMA- b -PEO- b -PMA was synthesized by the combination of atom transfer radical polymerization (ATRP) and Keck allylation [28] and was subsequently cyclized via metathesis polymer cyclization [29] using the second-generation Hoveyda–Grubbs catalyst in toluene to yield relevant cyclic PMA- b -PEO. The conversion of the allyl groups into the inner olefin unit through metathesis polymer cyclization was confirmed by 1 H NMR ( Supplementary Fig. S1 ), and a decrease in the hydrodynamic volume was observed by size exclusion chromatography, SEC ( Supplementary Fig. S2 ). These results demonstrate the formation of a cyclized structure. The obtained amphiphilic block copolymers were self-assembled in water to form micelles ( Fig. 1 ). The average values of the D h distribution by volume for the micelles of linear PBA 5 - b -PEO 70 - b -PBA 5 ( 1a , M n (NMR)=600–3100–600) and cyclic PBA 9 - b -PEO 70 ( 2a , M n (NMR)=1200–3100) were 11 and 12 nm, respectively, with a narrow distribution, which was determined by dynamic light scattering, DLS (plots at a NaCl concentration of 0 mg ml −1 in Fig. 2 , Table 1 ). In addition, atomic force microscopy (AFM) showed that the self-assembled structures exhibited a spherical morphology with sizes consistent with the DLS results ( Supplementary Fig. S3 ). We attempted to vary the segment composition of the PBA–PEO amphiphiles to investigate the influence on the stability of the micelles. However, because of the strong hydrophobicity and/or steric hindrance of PBA, PBA 6 - b -PEO 73 - b -PBA 6 with M n (NMR) of 800–3200–800 and polydispersity index (PDI) of 1.18 did not form a micelle selectively. Instead, a precipitate (that is large agglomerates) was formed via phase separation under general self-assembly conditions (?0.5 mg ml −1 ), which suggests the need for a specific segment composition. However, we found that block copolymers with PMA segments can be self-assembled to afford a micelle in a relatively wide molecular weight range. Thus, linear PMA- b -PEO- b -PMA with M n (NMR) values of 1400–3200–1400 ( 1b ), 1100–3100–1100 ( 1c ) and 1100–2800–1100 ( 1d ) were synthesized and cyclized to produce 2600–3000 ( 2b ), 2600–3500 ( 2c ) and 1700–2900 ( 2d ), respectively ( Table 1 ). All of linear 1b – 1d and cyclic 2b – 2d gave a uniform micellar solution. On the other hand, linear PMA 36 - b -PEO 73 - b -PMA 36 with a M n value of 3100–3200–3100 precipitated by phase separation at 1.0 mg ml −1 . However, its cyclized product, PMA 71 - b -PEO 100 with a M n value of 6100–4400, formed a micelle, which was another topology effect, in which a cyclic polymer tends to form a self-assembled structure in comparison with a linear counterpart. The CMC was determined using the increased light scattering intensity method [20] , which revealed that linear 1b – 1d and cyclic 2b – 2d have analogous CMC values of ~0.1 mg ml −1 . The comparable size and morphology of the micelles were observed by AFM ( Supplementary Fig. S4 ). However, slightly larger average values of the D h distribution by number for linear PMA- b -PEO- b -PMA ( 1b , 1c , and 1d ; 16–19 nm) compared with those for cyclic PMA- b -PEO ( 2b , 2c , and 2d ; 13–14 nm) were determined using the DLS method ( Table 1 , Supplementary Fig. S5 ). In addition, static light scattering measurements showed larger N agg values for linear PMA- b -PEO- b -PMA ( 1b , 73; 1c , 75; 1d , 114) compared with those for cyclic PMA- b -PEO ( 2b , 63; 2c , 61; 2d , 79), as shown in Table 1 (ref. 30 ). Interestingly, the A 2 value, which accounts for the strength of the interaction between the dispersed particles or molecules in a solvent, for cyclic PMA- b -PEO (1.97 × 10 −4 –4.05 × 10 −4 ml mol g −2 ) was at least twofold greater than that of corresponding linear PMA- b -PEO- b -PMA (0.29 × 10 −4 –1.09 × 10 −4 ml mol g −2 ), as shown in Table 1 . This result suggests that the repulsive interaction between the micelles formed from linear PMA- b -PEO- b -PMA diminishes in comparison with that of cyclic PMA- b -PEO, which is most likely due to the presence of the intermicellar bridging [14] , [31] , [32] , [33] , [34] . 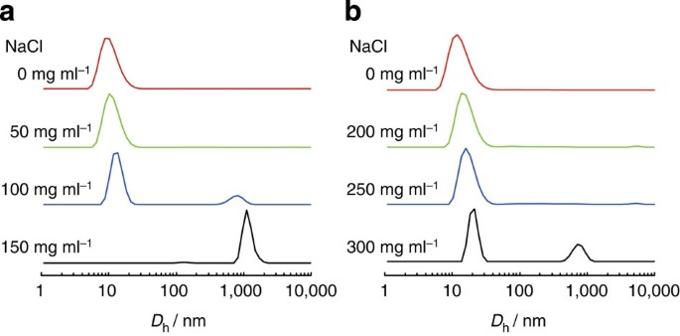Figure 2: NaCl concentration-dependentDhdistributions by volume determined by non-negative least squares analysis of the DLS data recorded at 25 °C. (a) Linear1aand (b) cyclic2a. The polymer concentration was 0.12 mM. The raw correlation data andDhdistributions by intensity and number are shown inSupplementary Fig. S6. Figure 2: NaCl concentration-dependent D h distributions by volume determined by non-negative least squares analysis of the DLS data recorded at 25 °C. ( a ) Linear 1a and ( b ) cyclic 2a . The polymer concentration was 0.12 mM. The raw correlation data and D h distributions by intensity and number are shown in Supplementary Fig. S6 . Full size image Table 1 Properties of micelles formed from linear and cyclic amphiphilic block copolymers. Full size table Cumulative salt and temperature-responsive micelles We observed the higher salt resistance of the micelle from cyclic 2a compared with that from linear counterpart 1a by measuring the respective C s values. Upon the stepwise addition of NaCl, the transmittance (%T) of the micellar solution of 1a started to decease at a NaCl concentration of 130 mg ml −1 at 25 °C ( Table 1 ). However, the solution that contained 2a remained transparent up to a NaCl concentration of 260 mg ml −1 . In the present study, C s and T c were defined by the salt concentration and temperature, respectively, at which the %T of a solution becomes 99% of the initial value. The turbidity results shown above should correspond to the transformation of the micelles to an agglomerate, and the change in the D h was monitored by DLS. At a NaCl concentration of 100 mg ml −1 for 1a ( Fig. 2a ) and 300 mg ml −1 for 2a ( Fig. 2b ), a peak at ~1 μm was visible in the D h distributions by volume. These salt concentrations indeed corresponded to those determined by the turbidity measurements. The raw correlation data and D h distributions by intensity and by number are shown in Supplementary Fig. S6 . The broad peak at around 200 nm in Supplementary Fig. S6c (0 and 50 mg ml −1 NaCl) and Fig. S6d (0, 200 and 250 mg ml −1 NaCl) could be due to equilibrated assemblies. However, these species are negligible in the D h distributions by volume ( Fig. 2 ) and by number ( Supplementary Fig. S6e and S6f ). In addition, the salted-out samples were observed using transmission electron microscopy (TEM) to confirm the formation of agglomerates because light scattering measurements are primarily governed by the larger particles in the specimen, which does not exclude the possibility that smaller particles still exist in significant amounts. The TEM images of the dried samples of 1a at 200 mg ml −1 NaCl ( Supplementary Fig. S7a ) and 2a at 300 mg ml –1 NaCl ( Supplementary Fig. S7b ) showed D h distributions that were consistent with the light scattering results, and the samples did not contain significant amounts of non-agglomerated micelles. On the basis of these results, the cyclic topology of the polymeric components exerts a decisive influence on the salt stability of the self-assembled products. Subsequently, we performed systematic studies to investigate the topology effects on the salt and thermal stability using both the PBA–PEO and PMA–PEO amphiphiles, the latter of which allowed us to prepare block copolymers with several different segment compositions. Therefore, the T c values of the respective micelles from the two types of block copolymers were determined at various NaCl concentrations (PBA–PEO, Fig. 3 ; PMA–PEO, Fig. 4 , Supplementary Fig. S8 , and Supplementary Fig. S9 ). As previously reported [23] , [35] , [36] , [37] , an increase in the temperature and salt concentration destabilizes a micellar entity in an interexchangeable manner because these two stimuli have a cumulative effect on the chemical potential of the system. In the absence of a salt, the T c values were determined to be 39 and 56 °C for the micelles from linear PBA 5 - b -PEO 70 - b -PBA 5 ( 1a ) and cyclic PBA 9 - b -PEO 70 ( 2a ), respectively, at a polymer concentration of 0.12 mM ( Table 1 ). When NaCl was added to the respective micellar solutions, a gradual decrease in the T c values was observed ( 1a , T c =30, 28, 26, and 25 °C at NaCl concentrations of 30, 60, 90 and 120 mg ml –1 , respectively, in Fig. 3a ; 2 a , T c =49, 45, 40, 36, 30 and 25 °C at NaCl concentrations of 30, 60, 90, 120, 180 and 240 mg ml –1 , respectively, in Fig. 3b ). Therefore, at a constant NaCl concentration of 30 mg ml –1 , the salt stability of the micelle increased from 30 °C ( 1a ) to 49 °C ( 2a ) via cyclization of the amphiphile. The result of the salt concentration–temperature experiments showed that the micelle from 2a is consistently more stable than that from 1a under the examined conditions ( Fig. 3c ). 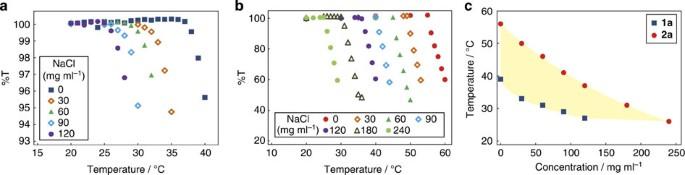Figure 3: Temperature-dependent turbidity measurements of micellar solutions under various NaCl concentrations. (a) Linear1aand (b) cyclic2aat a polymer concentration of 0.12 mM. The measurements were performed up to a temperature that was several degrees higher than the respectiveTcvalues. (c) Plots of temperature as a function of salt concentration for the cloud points of the micelles from linear and cyclic PBA–PEO block copolymers (blue square, linear1aand red circle, cyclic2a). Figure 3: Temperature-dependent turbidity measurements of micellar solutions under various NaCl concentrations. ( a ) Linear 1a and ( b ) cyclic 2a at a polymer concentration of 0.12 mM. The measurements were performed up to a temperature that was several degrees higher than the respective T c values. ( c ) Plots of temperature as a function of salt concentration for the cloud points of the micelles from linear and cyclic PBA–PEO block copolymers (blue square, linear 1a and red circle, cyclic 2a ). 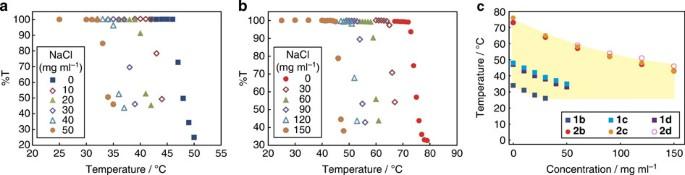Figure 4: Temperature-dependent turbidity measurements of micellar solutions under various NaCl concentrations. (a) Linear1dand (b) cyclic2dat a polymer concentration of 0.12 mM. The measurements were performed up to a temperature that was several degrees higher than the respectiveTcvalues. (c) Plots of temperature as a function of salt concentration for the cloud points of the micelles from linear and cyclic PMA–PEO block copolymers (blue square,1b; light blue square,1c; purple square,1d; red circle,2b; orange circle,2c; and pink open circle,2d). Full size image Figure 4: Temperature-dependent turbidity measurements of micellar solutions under various NaCl concentrations. ( a ) Linear 1d and ( b ) cyclic 2d at a polymer concentration of 0.12 mM. The measurements were performed up to a temperature that was several degrees higher than the respective T c values. ( c ) Plots of temperature as a function of salt concentration for the cloud points of the micelles from linear and cyclic PMA–PEO block copolymers (blue square, 1b ; light blue square, 1c ; purple square, 1d ; red circle, 2b ; orange circle, 2c ; and pink open circle, 2d ). Full size image Furthermore, a series of linear PMA- b -PEO- b -PMA and cyclized PMA- b -PEO with various segment compositions were examined to investigate the topology effects on the salt and thermal stability. The T c values of the micelles from linear 1b and cyclic 2b were determined to be 34 and 73 °C, respectively. Analogous to the PBA–PEO copolymers, a gradual decrease in the T c values was observed upon addition of NaCl ( 1b , T c =31, 28 and 26 °C at NaCl concentrations of 10, 20 and 30 mg ml –1 , respectively, in Supplementary Fig. S8a ; 2b , T c =64, 57, 52, 47, 43, 39, 36, 33 and 30 °C at NaCl concentrations of 30, 60, 90, 120, 150, 180, 210, 240 and 270 mg ml –1 , respectively, in Supplementary Fig. S8b ). Therefore, at a constant NaCl concentration of 30 mg ml –1 , the salt stability of the micelle from the PMA–PEO copolymer was enhanced from 26 °C ( 1b ) to 64 °C ( 2b ) by cyclization. In addition, the DLS profiles at 30 °C with an increasing NaCl concentration also showed steep increases in the z -average diameter at 20 mg ml –1 for 1b and at 280 mg ml –1 for 2b ( Supplementary Fig. S10 ), which were consistent with the decreases in %T determined from the turbidity measurements ( Supplementary Fig. S8 ). The D h distribution by number was not determined by non-negative least squares analysis here due to scattering caused by the large agglomerate. The results of the salt concentration–temperature experiments demonstrated that heating and the addition of a salt to the PMA–PEO copolymers ( 1b and 2b in Fig. 4c ) induced effects analogous to those observed in the case of the PBA–PEO copolymers ( 1a and 2a in Fig. 3c ). The above discussed results indicate that the topology effects of the salt and thermal stability have a certain degree of generality for the chemical structure of the hydrophobic segments. Next, we compared the salt and thermal resistance of micelles from linear ( 1c and 1d ) and cyclic ( 2c and 2d ) PMA–PEO copolymers with various segment compositions ( Table 1 ). In the previous report [14] , the T c values of micellar solutions of linear PBA 5 - b -PEO 64 - b -PBA 5 ( M n =700–2800–700) and cyclic PBA 11 - b -PEO 64 ( M n =1400–2800) were 24 and 73 °C, respectively, at a polymer concentration of 0.12 mM. However, the PDI of the PBA segments was expected to be high for the mean value of five repeating units, which led to the formation of asymmetric amphiphiles. For example, only two or three units were on one end, whereas the other end contained seven or eight units. Coupled with the limitation in accuracy to determine the low molecular weight of the segments by NMR, the difference in the T c values appeared between the previous and present studies. Therefore, the segment composition dependence of T c values was investigated using the PMA–PEO block copolymers, which had relatively longer hydrophobic segments, to avoid these issues. The results of the turbidity measurements are shown in Fig. 4a , and Supplementary Fig. S9 , and the plots of the temperature as a function of salt concentration are appended to the results of 1b and 2b in Fig. 4c . Copolymers 2c and 2d exhibited greater thermal and salt stability than did 1c and 1d , which is supported by higher A 2 values for 2c (4.05 × 10 –4 ml mol g –2 ) and 2d (1.97 × 10 –4 ml mol g –2 ) compared with those of 1c (1.04 × 10 –4 ml mol g –2 ) and 1d (1.09 × 10 –4 ml mol g –2 ), as shown in Table 1 . Therefore, the cyclic topology endowed the micelles with higher thermal and salt stability (Δ T c =26–39 °C at no addition of salt, Δ C s =140–260 mg ml –1 NaCl depending on the temperature) in the experimental segment composition range. On the basis of the segment composition dependence within linear PMA- b -PEO- b -PMA, 1b , which had a relatively higher molecular weight of the hydrophobic segments, exhibited a T c value (34 °C) lower than those of 1c (48 °C) and 1d (47 °C), as shown in Table 1 . This result is consistent with the A 2 value of 1b (0.29 × 10 –4 ml mol g –2 ) being less than one-third those of 1c (1.04 × 10 –4 ml mol g –2 ) and 1d (1.09 × 10 –4 ml mol g –2 ), which indicates a less-repulsive interaction for 1b arising from the longer PMA segments that tend to bridge micelles to form an agglomerate. However, the A 2 value of 2c (4.05 × 10 –4 ml mol g –2 ) was twice that of 2b (2.07 × 10 –4 ml mol g –2 ); this difference indicates a stronger repulsion between micelles and a slight increase in the T c values ( 2b , 73 °C and 2c , 76 °C), which is most likely due to the longer PEO segment of 2c with a nearly identical PMA length. Therefore, the effect of the hydrophobic segments appeared to be stronger than that of the hydrophilic segment. Nevertheless, the topology effects on the T c and A 2 values by the linear-to-cyclic conversion were more significant than the influences of the segment composition. Micelles with tuneable salt resistance The micelles formed from both types of cyclic block copolymers showed significantly greater salt stability under the experimental conditions ( vide supra ). We have previously shown that the tuning of the thermal stability of a micelle over a wide range can be achieved by coassembling linear and cyclic amphiphiles with distinct individual T c values [14] . Now, we have devised micelles with dually tuneable thermal/salt resistance. To demonstrate the tuneable salt stability, three micellar solution samples were prepared from various mixing ratios of linear 1a and cyclic 2a (75%/25%, 50%/50%, and 25%/75%), which were subjected to turbidity measurements by the addition of NaCl. The C s value of the coassembled micelles increased in proportion to the relative content of 2a (170 mg ml –1 at 25%, 190 mg ml –1 at 50% and 220 mg ml –1 at 75% in Fig. 5a ). 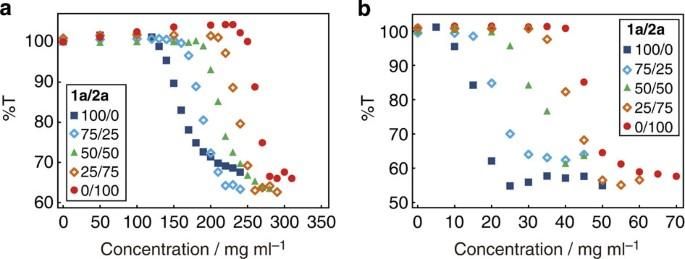Figure 5: Salt concentration-dependent turbidity measurements of micellar solutions of linear 1a, cyclic 2a, and their coassemblies at 25 °C. (a) NaCl and (b) MgSO4were used as a salt. The mixing ratio (1a/2a) was 100%/0%, 75%/25%, 50%/50%, 25%/75% and 0%/100%, and the total polymer concentration in a sample was 0.12 mM. Figure 5: Salt concentration-dependent turbidity measurements of micellar solutions of linear 1a, cyclic 2a, and their coassemblies at 25 °C. ( a ) NaCl and ( b ) MgSO 4 were used as a salt. The mixing ratio ( 1a / 2a ) was 100%/0%, 75%/25%, 50%/50%, 25%/75% and 0%/100%, and the total polymer concentration in a sample was 0.12 mM. Full size image In addition, we examined the tuneable salt resistance against MgSO 4 for the micelles from linear 1a and cyclic 2a, as well as their coassemblies. MgSO 4 was chosen because the salt is a typical component of permanent hard water and has a high salting-out capability. First, upon the stepwise addition of MgSO 4 to micellar solutions of 1a and 2a , a remarkable enhancement in the salt resistance of the cyclized amphiphile was observed. Therefore, the %T value of the micellar solution of 1a started to diminish at a MgSO 4 concentration of 10 mg ml –1 ( Fig. 5b , blue solid square). However, the solution of 2a remained transparent up to 45 mg ml –1 of MgSO 4 ( Fig. 5b , red solid circle). Therefore, the salt resistance was improved by a factor of two for NaCl and by more than a factor of four for MgSO 4 upon cyclization of the polymer amphiphile. In addition, three micellar solutions were prepared from a mixture of 1a and 2a (75%/25%, 50%/50% and 25%/75%) and were subjected to turbidity measurements with MgSO 4 . As observed with NaCl, the C s value of the coassembled micelles against MgSO 4 increased in proportion to the relative content of 2a (15 mg ml –1 at 25%, 25 mg ml –1 at 50% and 35 mg ml –1 at 75% in Fig. 5b ). On the basis of these experiments that show the cumulative topology effects for salt, as well as the thermal stability, the cloud points can be easily tuned through the coassembly of linear and cyclic block copolymers for the range of salt concentration and temperature shown in Figs 3c and 4c . Cumulative topology effects for micellar catalysis To exploit the topology effects, micellar catalysis [38] of a halogen exchange reaction (Finkelstein reaction) in water was conducted. A water-insoluble substrate, 1-(bromoacetyl)pyrene (41 mg, 0.13 mmol), was suspended in an aqueous NaCl solution (10 ml) in the presence of either a linear or cyclic amphiphile (0.12 mM, 1.2 μmol, 0.92 mol% of the substrate), as well as in the absence of them to produce 1-(chloroacetyl)pyrene. Initially, we used a NaCl concentration of 30 mg ml –1 at 45 °C, under which conditions the structure of the micelle from cyclic PBA- b -PEO 2a should persist but that from linear PBA- b -PEO- b -PBA 1a would not ( Fig. 3c ). However, only low conversion (<5% at 3 h) for both 1a and 2a with a marginal difference was observed. Therefore, the NaCl concentration and temperature were increased to 150 mg ml –1 and 60 °C, respectively, to stimulate the catalysis. As shown in Fig. 6a , 2a significantly accelerated the reaction (16% at 1 h, 28% at 3 h and 61% at 5 h; see also Supplementary Fig. S12 ) compared with 1a (12% at 1 h, 16% at 3 h and 41% at 5 h; see also Supplementary Fig. S11 ). Although we attempted to perform calculations of the rate constants of the reaction, the kinetics of micellar catalysis in a multiphase system is complicated and beyond the focus of this paper [39] . In contrast, essentially no product was formed in the absence of the copolymers ( Supplementary Fig. S13 ). These results are in agreement with the fact that 2a formed an aggregate with D h of ~10 nm even at 65 °C with a 150 mg ml –1 NaCl concentration, as shown in the temperature-dependent DLS measurements ( Fig. 6c ). The aggregate was most likely a micelle that encapsulated 1-(bromoacetyl)pyrene as a guest, which offers a large hydrophilic–hydrophobic interface area for an efficient reaction. In contrast, 1a afforded an agglomerate with a size of ~1 μm, which had a limited interface area for catalysis, at 55 °C and higher temperatures under the identical NaCl and 1-(bromoacetyl)pyrene conditions ( Fig. 6b ). The observed increase in stability of both micelles from 1a and 2a was presumably caused by the inclusion of the guest molecules in the core to promote the attractive interaction of the hydrophobic segments [40] , [41] . 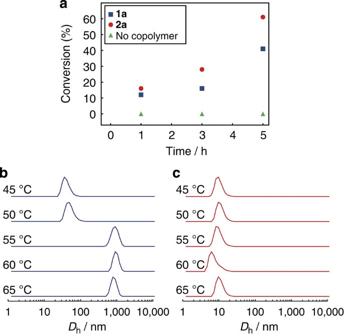Figure 6: Halogen exchange reaction of 1-(bromoacetyl)pyrene in an aqueous NaCl solution (150 mg ml–1). (a) Time-dependent conversion plots at 60 °C with and without the presence of linear1aor cyclic2aat a polymer concentration of 0.12 mM. Temperature-dependentDhdistributions by number determined by non-negative least squares analysis of the DLS data of (b) linear1aand (c) cyclic2a. Figure 6: Halogen exchange reaction of 1-(bromoacetyl)pyrene in an aqueous NaCl solution (150 mg ml – 1 ). ( a ) Time-dependent conversion plots at 60 °C with and without the presence of linear 1a or cyclic 2a at a polymer concentration of 0.12 mM. Temperature-dependent D h distributions by number determined by non-negative least squares analysis of the DLS data of ( b ) linear 1a and ( c ) cyclic 2a . Full size image Likewise, the halogen exchange reaction in the presence of linear PMA- b -PEO- b -PMA 1d or cyclic PMA- b -PEO 2d was performed to investigate the effects of the chemical structure of the hydrophobic segments. The conversion was ~10% at 3 h for both 1d and 2d at 150 mg ml –1 NaCl and 60 °C. The reaction was extended to 24 h; however, no significant difference between the linear and cyclic amphiphiles was observed. The temperature-dependent DLS measurements with a NaCl concentration of 150 mg ml –1 indicated that 1d formed a micrometre-order agglomerate even at 25 °C ( Supplementary Fig. S14b ). However, the size of the aggregate from 2d was ~20 nm at temperatures up to 45 °C and then suddenly increased to a micrometre scale at 55 °C ( Supplementary Fig. S14 ), which was consistent with the temperature-dependent turbidity measurements shown in Fig. 4b . Therefore, no stabilization effect by 1-(bromoacetyl)pyrene was observed for the micelles from 2d compared with those from 1a and 2a , which was most likely due to the strength of the interaction between the guest molecules and the core-forming hydrophobic segments. Despite the longer segment, the lower hydrophobicity of PMA compared with PBA was not sufficient to support the micellar structure by incorporating the guest molecules into the core under the catalytic conditions. Based on these results, the formation and retention of the micellar structure aided in the acceleration of the catalysis by offering a large interface area for reaction sites. Therefore, the micelle from 2a , which withstood the harsh reaction conditions (150 mg ml –1 NaCl, 60 °C), resulted in an enhanced catalytic activity through the collective topology effects of the higher resistance to the salt concentration and temperature, as well as the stabilization of the micelle core by the incorporation of the hydrophobic guest molecules. We describe below the observed remarkable topology effects on the salt resistance of the micelles from the cyclic amphiphiles by taking into account previous reports on associative ABA triblock copolymers [31] , [32] , [33] , [34] and our work on the enhanced thermal stability upon cyclization ( Fig. 7 ) (ref. 14 ). In a micellar solution, a dissolved electrolyte attracts and removes water molecules from the hydrophilic segment of the amphiphile at the interface of the micelle. Thermodynamically, dehydration is expected to take place predominantly at the PEO units located close to the hydrophobic segments rather than at those at the inner position of the hydrophilic segment [22] . For the micelles from the linear amphiphiles ( Fig. 7a , Stage I), one end of the folded polymer chain is promoted to leave the core due to thermal motion. When dehydration of the PEO units that are close to the hydrophobic segment of the free chain end occurs ( Fig. 7a , Stage II), the hydrophobicity of the moiety increases, and the moiety tends to move into the core of another micelle, which leads to intermicellar bridging ( Fig. 7a , Stage III) (refs 14 , 33 , 34 ). Eventually, a bridging network among the micelles develops and forms an agglomerate ( Fig. 7a , Stage IV). However, relevant segmental motions in the micelles from the cyclic amphiphiles are topologically prohibited to circumvent bridging ( Fig. 7b ), which results in significant enhancement of the stability against salt (dehydration) and heating (the thermal motion of chain ends). On the basis of the tuneable thermal/salt resistance of the coassembled micelles, the bridging is expected to occur statistically in proportion to the relative content of the linear amphiphile to gradually change the T c and C s values. 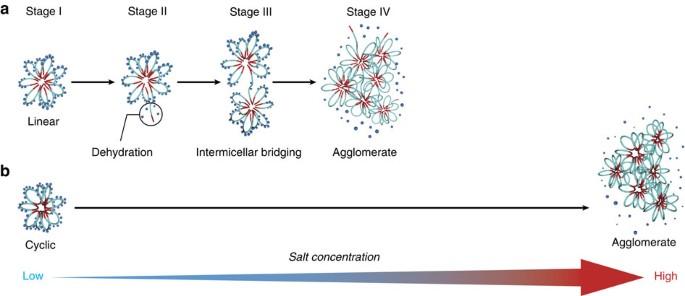Figure 7: Schematic representation for the proposed mechanism of agglomeration. The salt stability of a micelle formed from a cyclic amphiphilic block copolymer was enhanced in comparison with its linear counterpart likely as follows. (a) For a micelle from a linear amphiphile (Stage I), one end of the folded polymer chain is promoted to leave the core due to thermal motion. When dehydration of the PEO units that are close to the hydrophobic segment of the free chain end occurs (Stage II), the hydrophobicity of the moiety increases, and the moiety tends to move into the core of another micelle, which leads to intermicellar bridging (Stage III). Eventually, a bridging network among the micelles develops and forms an agglomerate (Stage IV). (b) On the other hand, relevant segmental motions in a micelle from a cyclic amphiphile are topologically prohibited to circumvent bridging. Figure 7: Schematic representation for the proposed mechanism of agglomeration. The salt stability of a micelle formed from a cyclic amphiphilic block copolymer was enhanced in comparison with its linear counterpart likely as follows. ( a ) For a micelle from a linear amphiphile (Stage I), one end of the folded polymer chain is promoted to leave the core due to thermal motion. When dehydration of the PEO units that are close to the hydrophobic segment of the free chain end occurs (Stage II), the hydrophobicity of the moiety increases, and the moiety tends to move into the core of another micelle, which leads to intermicellar bridging (Stage III). Eventually, a bridging network among the micelles develops and forms an agglomerate (Stage IV). ( b ) On the other hand, relevant segmental motions in a micelle from a cyclic amphiphile are topologically prohibited to circumvent bridging. Full size image In conclusion, self-assembled micelles were found to exhibit a remarkably higher salt tolerance due to cyclization of the polymeric amphiphiles. The dependence of the topology effects on the chemical structure and segment composition was also studied. We found that the stability of the micelles is reflected in the A 2 values and can be primarily attributed to the topology of the amphiphiles. Furthermore, the micelles formed from the cyclic amphiphiles had higher cumulative thermal/salt stability under the experimental conditions tested compared with their linear counterparts. The C s value was readily tuneable by changing the mixing ratio of the linear and cyclic amphiphiles during the coassembly. The enhanced salt- and thermo-resistant properties were exploited in micellar catalysis. As the improvement and control of the performance of polymeric materials normally require modification of the chemical structure, molecular weight and/or segment composition [42] , the reported topology effects provide a novel method for the design of highly functional materials and dual-stimuli-responsive systems [43] , [44] , [45] . Materials All commercial reagents were used as received unless otherwise noted. Tetrahydrofuran (THF) was distilled over Na wire. Linear PBA 5 - b -PEO 70 - b -PBA 5 ( 1a ) and cyclic PBA 9 - b -PEO 70 ( 2a ) were synthesized according to a previously reported procedure [10] . Thus, linear 1a was prepared from a bromoisobutyryl-terminated bifunctional PEO macroinitiator ( M n (NMR)=3100) via ATRP followed by Keck allylation [28] , [46] . Subsequently, allyl-telechelic 1a was cyclized to yield 2a in the presence of the second-generation Grubbs catalyst in dilution ( Fig. 1 ). Synthesis of linear PMA- b -PEO- b -PMA (1b, 1c and 1d) In a typical procedure, allyl-telechelic PMA 13 - b -PEO 64 - b -PMA 13 ( 1d ) was prepared through ATRP and subsequent Keck allylation [28] , [46] . The bromoisobutyryl-terminated bifunctional PEO macroinitiator (1.0 g, 0.31 mmol, M n (NMR)=3100), methyl acrylate (4.8 g, 56 mmol), 2,2′-bipyridyl (290 mg, 1.9 mmol) and CuBr (90 mg, 0.62 mmol) were placed in a test tube, and the resulting suspension was degassed by three freeze–pump–thaw cycles. The test tube was sealed under vacuum, and the suspension was stirred at 90 °C for 5 min. The reaction mixture was quenched in liquid nitrogen and allowed to warm to room temperature. After the remaining methyl acrylate was removed under reduced pressure, toluene (5 ml) and allyltributyl stannane (0.96 ml, 3.1 mmol) were added to the residue, and the resulting suspension was degassed by three freeze–pump–thaw cycles. The test tube was sealed under vacuum, and the suspension was stirred at 110 °C for 18 h. The reaction mixture was precipitated in n -hexane and was filtered through a plug of alumina using THF as an eluent. The filtrate was concentrated and reprecipitated in n -hexane to allow isolation of 1d as a waxy solid (877 mg) in 57% yield. M n (NMR)=1100–2800–1100 for PMA 13 - b -PEO 64 - b -PMA 13 , M p (peak molecular weight by SEC calibrated with polystyrene standards)=6,000, PDI=1.23. 1 H NMR: δ (p.p.m.) 1.14–1.18 (t, 12H, –C(C H 3 ) 2 –), 1.48–2.15 (m, –C H 2 CH(CO 2 CH 3 )–), 2.20–2.50 (m, –CH 2 C H (CO 2 CH 3 )–), 3.42–3.89 (m, –OC H 2 C H 2 O–, –OC H 2 CH 2 OC(=O)–, –CO 2 C H 3 ), 4.20 (m, 4H, –OCH 2 C H 2 OC(=O)–), 5.04 (m, 4H, –CH 2 CH=C H 2 ), 5.68 (m, 2H, –CH 2 C H =CH 2 ). Linear 1b and 1c were synthesized following a similar procedure. Synthesis of cyclic PMA- b -PEO (2b, 2c and 2d) In a typical procedure, the second-generation Hoveyda–Grubbs catalyst (70 mg, 0.11 mmol) was added to a toluene solution of allyl-telechelic 1d (0.25 g l –1 , 800 ml), and the resulting solution was stirred at 80 °C for 24 h. Ethyl vinyl ether (30 ml) was added to the reaction mixture to quench the catalyst. The colour of the solution immediately changed from brown–green to brown. The mixture was further stirred at 80 °C for 16 h. The reaction mixture was concentrated and subjected to silica gel column chromatography. The byproducts and impurities were first eluted with EtOAc, and the product was collected with MeOH. The crude product was fractionated by preparative SEC with CHCl 3 as an eluent at a flow rate of 3.5 ml min –1 to allow isolation of 2d (161 mg) in 81% yield. M n (NMR)=1700–2900 for PMA 20 - b -PEO 66 , M p =4800, PDI=1.20. 1 H NMR: δ (p.p.m.) 1.13–1.17 (t, 12H, –C(C H 3 ) 2 –), 1.50–2.15 (m, –C H 2 CH(CO 2 CH 3 )–), 2.20–2.52 (m, –CH 2 C H (CO 2 CH 3 )–), 3.42–3.95 (m, –OC H 2 C H 2 O–, –OC H 2 CH 2 OC(=O)–, –CO 2 C H 3 ), 4.18 (m, 4H, –OCH 2 C H 2 OC(=O)–), 5.32 (m, 2H, –C H =C H –). Cyclic 2b and 2c were synthesized following a similar procedure. The difference in the molecular weights of the linear prepolymers and the corresponding cyclic products was caused by column chromatography and preparative SEC fractionation. Small portions of the product were removed along with byproducts and impurities during the purification, resulting in the slight change in M n (NMR). Preparation of aqueous micellar solutions Aqueous micellar solutions of the PBA–PEO block copolymers (linear 1a and cyclic 2a ) were prepared via the solvent evaporation method according to a previously published protocol [47] . Thus, distilled water (10 ml) was added to a vigorously stirred THF solution of 1a or 2a (2.3 mM, 1.0 ml) at a rate of one drop per 5 s. THF was removed from the mixture with a rotary evaporator, and the remaining aqueous solution was diluted with distilled water to a total volume of 10 ml to yield a 0.23-mM micellar solution. The preparation of micellar solutions from the PMA–PEO block copolymers (linear 1b – d and cyclic 2b – d ) was performed via the direct dissolution method [48] using ultrasound because of the moderate hydrophobicity of the PMA segments compared with that of the PBA counterparts. Thus, in a typical procedure, 1b (10 mg) and distilled water (10 ml) were placed in a vial, and ultrasound was applied to form a homogeneous micellar solution. The direct dissolution method was also attempted to self-assemble 1a and 2a . However, likely because of the strong hydrophobicity of the PBA segments and the formation of a network structure in the solid state, 1a was not taken up in water by ultrasound. Halogen exchange reaction NaCl (0.30 or 1.50 g) was added to a micellar solution (0.12 mM, 10 ml) of linear PBA 5 - b -PEO 70 - b -PBA 5 ( 1a ), linear PMA 13 - b -PEO 64 - b -PMA 13 ( 1d ), cyclic PBA 9 - b -PEO 70 ( 2a ) or cyclic PMA 20 - b -PEO 66 ( 2d ), and the resulting mixture was stirred at 45 or 60 °C. The substrate, 1-(bromoacetyl)pyrene (41 mg, 0.13 mmol), was added to initiate catalysis. A portion (1 ml) of the reaction mixture was sampled out at given reaction times and added to CHCl 3 (2 ml) to extract the product, 1-(chloroacetyl)pyrene, as well as the unreacted substrate. The organic phase was separated and dried under reduced pressure. The conversion was determined by the ratio between the 1 H NMR peak areas of the chloroacetyl (4.96 p.p.m.) and bromoacetyl groups (4.75 p.p.m.) ( Supplementary Figs S11 and S12 ). In addition, the halogen exchange reaction in the absence the block copolymers was performed as a control experiment ( Supplementary Fig. S13 ). NMR measurements 1 H NMR spectra were recorded on a JEOL JNM-AL300 spectrometer operated at 300 MHz. CDCl 3 was used as the solvent, and the chemical shifts were reported relative to the signal of tetramethylsilane. The M n (NMR) values were determined by end-group analysis. SEC measurements SEC measurements were performed on a Tosoh model CCPS equipped with a refractive index detector (model RI 8020) and a TSK G3000HXL column. THF was used as the eluent at a flow rate of 1.0 ml min –1 . Light scattering measurements DLS and static light scattering measurements were performed on a Malvern Zetasizer Nano spectrometer equipped with a He–Ne laser ( λ =532 nm). The light scattering signal was obtained at a fixed angle of 173°. Non-negative least squares [49] , [50] , [51] , [52] and cumulants analyses provided in software built into the instrument were used to determine the D h distributions and z -average diameter, respectively. N agg and A 2 were determined by Debye plots with polymer concentrations of 10, 5.0, 2.5, 1.0 and 0.50 mg ml –1 . The d n /d c values were calculated based on the weight fractions of the segments [53] , where the d n /d c values of the homopolymers are 1.47 (ref. 54 ) for PBA and PMA and 1.45 (ref. 55 ) for PEO. For the temperature-dependent measurements under the micellar catalysis conditions ( Fig. 6b , and Supplementary Fig. S14 ), the specimens were prepared as follows. NaCl (150 mg) and 1-(bromoacetyl)pyrene (4.0 mg) were added to a micellar solution of 1a , 1d , 2a or 2d (0.12 mM, 1.0 ml) under vigorous stirring. Undissolved 1-(bromoacetyl)pyrene, which disturbs light scattering, was filtered off with a 0.45-μm membrane filter before the measurements. Turbidity measurements The transmittance of a micellar solution was measured at 600 nm on a JASCO Ubest V-560 spectrophotometer. For Fig. 3a , Fig. 4a , Supplementary Fig. S8 and Supplementary Fig. S9 , %T value was recorded immediately after the temperature reached a set value. For Fig. 5 , %T value was recorded after the addition of NaCl or MgSO 4 and after the mixture was stirred for 3 min. AFM observations A few drops of a 0.5 or 1.0 mg ml –1 micellar solution were placed onto a silicon substrate and blown away with a blower. AFM observations of the residual sample on the substrate were performed on a Seiko SPA400 microscope operated in DFM mode. TEM observations A few drops of a 0.5 mg ml –1 micellar solution precipitated by the addition of NaCl were placed onto a carbon-coated Formvar TEM grid and blown away with a blower. TEM observations were performed on a Hitachi H-7650 Zero A microscope operated at 75 kV. How to cite this article: Honda, S. et al. Tuneable enhancement of the salt and thermal stability of polymeric micelles by cyclized amphiphiles. Nat. Commun. 4:1574 doi: 10.1038/ncomms2585 (2013).